The uncertainty principle enables non-classical dynamics in an interferometer The quantum uncertainty principle stipulates that when one observable is predictable there must be some other observables that are unpredictable. The principle is viewed as holding the key to many quantum phenomena and understanding it deeper is of great interest in the study of the foundations of quantum theory. Here we show that apart from being restrictive, the principle also plays a positive role as the enabler of non-classical dynamics in an interferometer. First we note that instantaneous action at a distance should not be possible. We show that for general probabilistic theories this heavily curtails the non-classical dynamics. We prove that there is a trade-off with the uncertainty principle that allows theories to evade this restriction. On one extreme, non-classical theories with maximal certainty have their non-classical dynamics absolutely restricted to only the identity operation. On the other extreme, quantum theory minimizes certainty in return for maximal non-classical dynamics. The uncertainty principle has been the subject of much discussion since the early days of quantum theory [1] , [2] . It is a quintessentially quantum phenomenon in the sense that in classical probability theory there is no ban on systems where all quantities can be deterministically known. A deeper understanding of this principle is a key aim in quantum foundations, believed to be holding the key to the understanding of a wide host of quantum phenomena. One important insight is that one may formulate theories similar to quantum theory, with the crucial difference that while there are measurements that cannot be measured at the same time, these are not subject to an uncertainty relation [3] , [4] . These theories can, as a direct consequence of having less (or even no) uncertainty, have more Bell violation than possible in quantum theory and may allow for greater work extraction than permitted by the second law of thermodynamics [3] , [5] , [6] , [7] . In these cases the uncertainty principle acts as a fundamental limiting factor. To formulate such possibly non-quantum theories it is natural to use the convex framework for probabilistic theories [4] , [8] , [9] , [10] , [11] , [12] , [13] , as essentially any experiments yielding tables of data can be formulated in this way [8] , [9] . Quantum theory is then but a special case in a wider set of theories. One is free to add or remove features from quantum theory and investigate the consequences. This approach has yielded interesting results in the fields of information theory [4] , statistical mechanics [11] and axiomizations of quantum theory [8] , [12] , [13] . Many non-classical quantum phenomena also involve the notion of phase. The state of a quantum particle is not uniquely specified by its probabilities of being found at different positions, but in addition one must also assign a phase to each position. This notion can be generalized to any probabilistic theory, and dynamics which change these phases are termed non-classical [14] . One physical set-up where such phases may be observed and manipulated is the Mach–Zehnder interferometer, as shown in Fig. 1 . (For discussions relating to interference in post-quantum theories in a different context see refs 15 , 16 , 17 .) 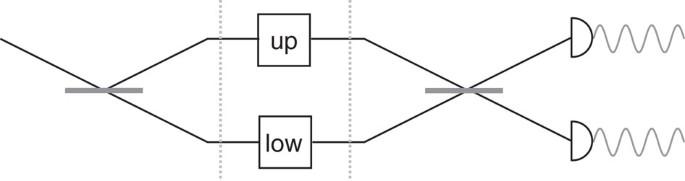Figure 1: The Mach–Zehnder interferometer. Branch locality, the restriction whose consequences the uncertainty principle enables escape from, states that if the (possibly post-quantum) particle is with probability 1 to be found in one of the branches of the interferometer (for example, up), then operations on the other spatially disjoint branch (for example, low) cannot change the operational state of the particle. Figure 1: The Mach–Zehnder interferometer. Branch locality, the restriction whose consequences the uncertainty principle enables escape from, states that if the (possibly post-quantum) particle is with probability 1 to be found in one of the branches of the interferometer (for example, up), then operations on the other spatially disjoint branch (for example, low) cannot change the operational state of the particle. Full size image In this present research, we see that transformations in an interferometer are heavily restricted by a principle forbidding action at a distance. We call this principle branch locality: the demand that if the system has no probability of being found in a particular region (for example, branch of an interferometer), then actions on that region cannot have an observable impact on the system. It turns out that in the quantum case, the non-classical transformations are entirely immune to this branch locality restriction and that the reason for this is the uncertainty principle. The mathematical argument is very similar to how a body sitting on a surface with total friction may still spin around if its shape is restricted such that it only has one point on the surface: sometimes one restriction can reduce the impact of another. We investigate this effect and show that it is an instance of a wider phenomenon. Branch locality does not impose any restrictions on non-classical dynamics in theories with something like the uncertainty relation. On the other extreme, theories with full certainty have any non-classical dynamics restricted to the identity operation by branch locality. One may say that quantum theory maximizes its non-classical dynamics at the expense of certainty. Overview We proceed by introducing the key concepts of the operational framework for probabilistic theories, such as states and transformations, as well as examples of theories, including quantum theory and the so-called box-world theory. We do this in the context of an interferometer, which is the physical scenario we focus on here. Then we define branch locality in that language. We show how in box-world, when there is no uncertainty between the position and other measurements, no state-changing transformations at all can exist without violating branch locality. We then consider why the proof does not go through in quantum theory, showing that this is due to the uncertainty relation. We demonstrate the general trade-off in theories between local dynamics and the amount of uncertainty. This discussion includes the introduction of a generalization of mutually unbiased bases. Finally, we discuss the implications, in particular, with regard to computation with different non classical theories. Interferometers in the convex probabilistic framework We start with the simplest quantum case and then generalize it. In the case of quantum theory one may describe an ideal Mach–Zehnder interferometer ( Fig. 1 ) using a single qubit, that is, a two-dimensional Hilbert space. The state after the first beam splitter can be expressed in the which-branch basis as | ψ ›= c up | z up ›+ c low | z low ›. The observable giving the expected position corresponds to Z = z up | z up ›‹ z up |+ z low | z low ›‹ z low | for some labels z up , z low that we assign to the respective branches. Here it will be convenient to label these ±1, respectively, so that the observable is modelled by the Pauli matrix Z =| z up ›‹ z up |−| z low ›‹ z low |. (The argument also works for labellings other than ±1.) The state space of a qubit can be represented by real vectors using the well-known Bloch sphere, see Fig. 2 . Here a state is represented by a real-valued vector of expectation values: [‹ X ›, ‹ Y ›, ‹ Z ›] T where X and Y are the other two Pauli matrices, and ‹ g ›= p ( g =+1)− p ( g =−1). 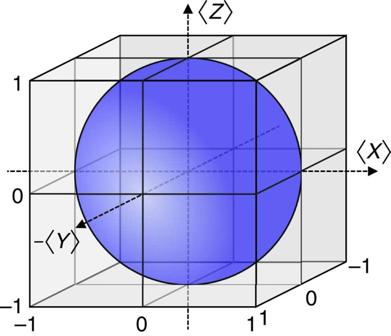Figure 2:State spaces. The quantum state space is the (Bloch) sphere. We also consider the possibility of other states outside the sphere. The case of the maximal cubic state space is an instance of the so-called ‘box-world’. The branch locality restriction mandates that states on the upper or lower plane are invariant under any transformation. The Bloch sphere, respecting the uncertainty principle, touches the cube at only one point on each face and is unrestricted in its dynamics, but the box-world cube is totally frozen. Mixtures of states correspond to probabilistic (convex) combinations of these states, lying inside the sphere of pure states defined by Figure 2: State spaces . The quantum state space is the (Bloch) sphere. We also consider the possibility of other states outside the sphere. The case of the maximal cubic state space is an instance of the so-called ‘box-world’. The branch locality restriction mandates that states on the upper or lower plane are invariant under any transformation. The Bloch sphere, respecting the uncertainty principle, touches the cube at only one point on each face and is unrestricted in its dynamics, but the box-world cube is totally frozen. Full size image The above equation constitutes an uncertainty relation; for example if ‹ Z ›=1 one must have ‹ X ›=‹ Y ›=0. The more familiar formulation in terms of standard deviations, that , is implied by equation (1) (recall that (Δ g ) 2 =‹ g 2 ›−‹ g › 2 ). The real vector used above amounts to an operational description of the state. One may now entertain the possibility of post-quantum states by associating them with points outside the sphere of pure quantum states. In the present representation of states, the state [1, 1, 1] T , for example, is not allowed in quantum theory as it violates the uncertainty principle of equation (1). We shall here a priori allow such states and later rule them out. In fact, we shall only a priori assume that the theory fits into the convex framework (essentially any experiment yielding a data table can be described in this manner [8] , [9] ). A key rule is that the state can be represented as a real vector s . A measurement is associated with a set of outcomes { e i }, each also represented by a real vector e i (known as an ‘effect’) such that the probability of each outcome e i for that measurement on a state s is given by the inner product, P ( e i )= e i · s . It will be crucial to our argument to consider the transformations of states. These must take all allowed states to allowed states. They must also respect the linearity of probabilistic mixtures: for a transformation T acting on a mixture of two states, ν 1 and ν 2 , we have T ( p 1 ν 1 + p 2 ν 2 )= p 1 T ( ν 1 )+ p 2 T ( ν 2 ). These transformations are real-valued matrices acting on state vectors, up to the subtlety that one should now add an extra component n to the state vector corresponding to the ‘normalization’ of the state ( n =1 for normalized states) in the expectation value representation. Phase transformations have been recently defined in this framework [14] , generalizing the idea of a phase plate in quantum theory. It was shown that a theory is classical (meaning it can be described by classical probability theory) if and only if it has no non-trivial phase transformations. We shall here refer to phase transformations with respect to the position measurement as non-classical transformations. A theory is specified by the set of states (which implicitly assumes a set of measurements and outcomes has been defined) and the allowed transformations. Following Hardy [8] we call sets of measurements whose statistics are sufficient to characterize any state in the given theory ‘fiducial’. For example, the Pauli matrices X , Y and Z are fiducial measurements for a qubit. As well as making general statements about all theories, we shall refer to three concrete examples. The quantum qubit case has states represented as ν =[ n , ‹ Z ›, ‹ X ›, ‹ Y ›] T . The allowed transformations consist of both reversible SO(3) transformations as well as linear transformations that shrink the sphere. Second, we shall call the case of a diagonal density matrix (such that, ‹ X ›=‹ Y ›=0) the classical case, modelled as ν =[ n , ‹ Z ›, 0, 0] T . Here any matrix preserving or shrinking the line of states is allowed. Finally, the maximal state space of all probabilistic mixtures of the corners [ n , ± n , ± n , …] T is known as the state space of a single system in the box-world. The special case of [ n , ± n , ± n ] T is termed a (2-in 2-out) ‘gbit’ [4] . This can (for n =1) be visualized as the square X – Z plane slice of the cube in Fig. 2 . Gbits are currently of great interest in the context of understanding whether there can be Popescu–Rohrlich (PR) boxes. These are hypothetical maximally Bell-violating systems (see ref. 3 ). The pure states of a gbit, the corners of the maximal state space, are the conditional marginal states of a PR box [4] in the same way that pure qubit states are related to Bell states. Thus if a PR box can exist then so can a gbit. In box-world, the allowed transformations on single systems are normally taken to be any matrix that preserves or shrinks the state space (but our arguments will apply even if one is not so permissive with the transformations). Branch locality restriction Branch locality, as described in Fig. 1 , can now be formalized as an operational principle. Definition 1: Principle of branch locality Physical actions on one region of space have no immediate effect on systems with no probability of being detected in that region. For an interferometer with many branches, we associate the effect with measuring the position to be within a subset of branches . Consider a state with no support in such that . When is acted on by a transformation , which is localized to , it must not change: In particular, if a system is in state ν b associated with a single branch b and we act on it with a transformation T b ′ on another branch b ′≠ b , then We shall also impose a more obvious condition on operations at different branches. We take the state to be described by someone without access to outcomes of any measurements performed on the local branches. Local transformations T acting on the respective branches must then not alter the statistics associated with the Z measurement. In the case of just two branches, using the Bloch sphere representation: if the transformation takes ‹ Z › to ‹ Z ›′ then this is simply written as In the language of ref. 14 this amounts to demanding that the transformation is a phase transformation associated with the position measurement Z . Moreover, we shall assume that each disjoint branch has at least one state where, if measured in the which-branch basis, the system will be found in that branch with certainty. We now show that in the extreme case of box-world where there is no uncertainty relation between position and other measurements, no transformations respect branch locality. Here in the main body we give a more pedagogical argument for the simplest case of box-world, describing a two-branch interferometer with a position measurement Z and one other measurement X defining a square state space. In the Methods we prove this statement for a more general case of box-world, and a wider class of related theories. Using the notation defined above, if we take a state to be in the upper branch with certainty, it must have the form ν up =[ n , n , ‹ X ›] T (recall that n is the state normalization with n =1 for a normalized state, and so ‹ Z ›= n for the upper branch). Consider the effect on this state by an operation on the lower branch. From the above considerations, equations (3) and (4) both hold. Recalling, moreover, that the transformation is a real matrix, it follows that: Consider the ranges of the different variables for gbits: n can take values in the range 0–1, and ‹ X › from − n to n (even when ‹ Z ›=± n , ‹ X › is free to take any value in this range). As T low is independent of the state it acts on, we can also consider the effect of T low on states where ‹ Z › takes other values in the range [− n , + n ], subject only to the restriction in equation (4), and the requirement that T low maps allowed states to allowed states. It follows with a little work that By considering states where ‹ Z ›=− n , we can similarly show that the only allowed transformations on the upper branch is T up =. Thus we see that all dynamics violate branch locality in the simplest case of box-world. We prove this statement for similar interferometers with any number of branches or measurements in the Methods. Uncertainty principle versus branch locality The above proof for a gbit does not carry through in quantum theory. The proof makes use of the fact that, for gbits, when ‹ Z ›=±1, ‹ X › is still free to take all possible values. This is a violation of the quantum uncertainty principle and a key difference between box-world and quantum theory. One may therefore think that the uncertainty relation renders the restriction of branch locality trivial. We shall prove a statement to this effect. We begin with some definitions that we will use to state our main result; these may also be of independent interest. Definition 2: Fully conditionally restricted A state space is fully conditionally restricted by a particular measurement if fixing any particular outcome of that measurement to occur with certainty is sufficient to completely specify the state. An important type of full conditional restriction is the kind that arises when a set of measurements are subject to the type of uncertainty relation that mutually unbiased quantum measurements (such as the Pauli matrices on a qubit) obey: Definition 3: Quantum-like uncertainty relation A set of measurements obey a quantum-like uncertainty relation if for every state where one of these measurement has an outcome that occurs with certainty, the outcomes of all other measurements in the set are governed by uniformly random distributions. Finally, we consider the opposite extreme to fully conditionally restricted sets of measurements. Definition 4: Fully independent A state space is fully independent of a given measurement if fixing the outcome of that measurement only reduces the number of degrees of freedom in the choice of state by the number of possible outcomes of the measurement. For example, consider a gbit (defined above) with two or more fiducial measurements. If one of these fiducial measurements is the position measurement, the other fiducial measurement(s) is fully independent of the position measurement. A state space can only be both fully conditionally restricted and fully independent of the position measurement if the position statistics uniquely specify the state. Otherwise there would be a contradiction. This special case corresponds to classical probability theory describing the measurement outcomes (under our assumption that each branch can be occupied with certainty). In this case there are no non-classical dynamics to be ruled out as there are no phase transformations [14] . With these definitions, we now state our main theorem: Theorem: If the state space is a fully restricted conditional on the position measurement, then any non-classical transformation can always be localized to a strict subset of branches without violating branch locality. If the state space is instead fully independent of the position measurement then no non-classical transformations (of form T≠) can be localized to any strict subset of branches without violating branch locality. An intuitive understanding may be reached on why the restriction placed by uncertainty enables non-classical dynamics: branch locality places a joint restriction on the states and transformations, and the restriction on transformations is weakened by strengthening the restriction on the set of states. A consequence of this for interferometers with state spaces fully independent of the position measurement is that no non-classical dynamics are possible even with access to operations on all but one branch. In interferometers that are fully conditionally restricted on the position measurement, such as when there is a quantum-like uncertainty relation between the position and the other fiducial measurements, this is not the case. Uncertainty and mutually unbiased measurements The main theorem contrasts the dynamics of interferometers conditionally restricted by the position measurement to those without restriction. We now make explicit the link between conditional restriction and uncertainty. Uncertainty, the idea that knowing more about one measurement means that another measurement is more random, is a special instance of a conditional restriction. In this section we show that the quantum uncertainty relation is the only possibly full conditional restriction for an important class of measurements, namely a generalization of mutually unbiased bases. An example to bear in mind is the qubit. Instead of representing the state in terms of the mutually unbiased Pauli matrices, as ν =[ n , ‹ Z ›, ‹ X ›, ‹ Y ›] T , we could have represented it as . In both cases, knowing the outcome of Z with certainty fully determines the statistics for the other measurements (that is, both sets of measurements are fully conditionally restricted), but only in the former case does the set of measurements obey the quantum-like uncertainty relation defined above. We can identify a specific set of measurements where full conditional restriction requires a quantum-like uncertainty relation: mutually unbiased measurements, a generalization of quantum mutually unbiased bases, which we now propose. Definition 5: Mutually unbiased measurements A set of measurements are mutually unbiased if for all allowed states, the outcome probabilities of one measurement in the set can be permuted to form another valid state without having to change the statistics of any other measurement in the set. When such a requirement is applied to projective measurements in quantum theory, it reduces to the standard definition of mutually unbiased bases. One sees from the definitions that any set of mutually unbiased measurements that is fully conditionally restricted obeys a quantum-like uncertainty relation, because only the uniform distribution is permutation-invariant. In this paper, we have demonstrated the importance of the uncertainty principle (and more generally, the conditional restrictions) for set-ups that are subject to locality requirements. The restriction placed by locality is so strong that without these other types of restrictions to mitigate its effects, absolutely no non-classical dynamics are admitted. One may say that uncertainty is the sacrifice that quantum theory makes to maximize its non-classical dynamics. One may think that the famous Aharonov–Bohm effect [18] brings branch locality into question, but in line with the standard interpetation of that effect, we view the procedure (for example, the switching on or off of a solenoid) as a many-branch operation (changing the potential on both occupied branches), so the resulting change in the interference pattern is not a violation of branch locality. Our introduction and consideration of the branch locality principle has more dramatic implications compared with previous results concerning the restricted dynamics in box-world [4] , [19] , [20] . When there is no uncertainty between position and the other measurements, we have ruled out any non-trivial dynamics, whether reversible or not, and by non-trivial we mean any transformation that is not the identity (whereas the word ‘trivial’ in the title of ref. 20 refers to the lack of correlating interactions). Moreover, we show that the same restriction holds for any interferometer in the convex framework with a state space fully independent of the position measurement, not just box-world. As any computation has to be performed as an evolution of a physical system, our results can be interpreted as saying that computation using a (two- or multi-branch) Mach–Zehnder interferometer is trivial when the state space is fully independent of the position. This experimental setting stands out as being the original setting in which quantum computation was conceived, with the Deutsch–Jozsa algorithm [21] arising naturally by considering what one can do with a quantum system in an interferometer. In ref. 22 it is argued that, more generally, key quantum algorithms can be viewed as a three-stage interferometer experiment: first, prepare a superposition of different branches; second, apply different phase shifts to different branches; and third, bring the branches together and make a measurement, yielding information about the phase shifts that were done. The apparent ability to prepare and individually address several inputs in the first and second stages is called quantum parallelism [21] (distinct from classical parallel computation). Our result suggests that adopting an uncertainty relation enables this parallelism, directing the search for post-quantum theories with stronger computational power to those that respect conditional restrictions such as the uncertainty relation, for example, ‘systems with limited information content’ [23] , [24] , [25] . The general probabilistic theory framework We first introduce the key concepts of the operationalist approach that we will use: the framework for general probabilistic theories also known as the convex framework. For a more detailed description of the framework see, for example, refs 8 , 13 . The framework is operational in the sense that essentially any experiment producing a data table can be described in this way [8] , [9] . For readers familiar with quantum theory it can also be helpful to think of the general probabilistic theory framework as a generalization of quantum theory. In quantum theory, there is a system that is prepared in a state ρ , determined by the preparation in question. There is a set of measurements one may do, each represented by a set of projection operators (or more generally positive-operator valued measure (POVM) elements). The operationally significant quantities, the probabilities of given outcomes, are given by P i =Tr( ρ Π i ). Viewed more abstractly, the state is a vector ρ in the vector space of Hermitian operators. A projection operator is also such a vector, Π say. In other words, we may pick a basis of the vector space and write ρ =∑ i ξ i e i and Π =∑ j ν j e j . (Examples of such bases are the Pauli operators and the pure state basis given by Hardy in ref. 8 .) Note that the coefficients of these expansions are real, so this is termed a real vector space. Tr( ρ Π) is then the Hilbert–Schmidt inner product (for Hermitian matrices), which we may write as ‹ ρ , Π ›. If the basis elements are chosen so that they are orthogonal with respect to the norm, and all having the same inner product c with themselves, we see that ‹ ρ , Π ›= ξ · ν c where the right hand side is the standard Euclidean norm. Thus, we may represent a quantum state, measurements on it, and the resulting probabilities in terms of real vectors and the Euclidean norm. In the framework, we more generally represent the state of a system s as a real vector, and the measurement–outcome pairs, called ‘effects’ for historical reasons, as real vectors e (for example, in the quantum case such a vector could be associated with X =+1, where X is the Pauli X ). The probability of the outcome associated with a given e is given by s · e . Part of the specification of a given theory is specifying which states and effects are allowed. All convex combinations (mixtures) of allowed states are always allowed, written as s =∑ i p i s i (hence the name ‘convex framework’). A state is said to be pure if it is not a non-trivial mixture of other states, otherwise it is called mixed. Transformations are represented as real matrices acting on the state vector (following from the requirement of respecting mixtures, see for example, ref. 8 ). They must take all allowed states to allowed states, but there may be further restrictions specified for a given theory in the framework. A transformation T is termed reversible if its inverse T −1 is also allowed in the theory. Following ref. 14 , we shall term transformations that leave the statistics for the designated position measurement-invariant for any state non classical dynamics. As well as quantum theory and theories contained therein (such as classical probability theory), one may also formulate a theory called box-world in this way. Box-world contains all states that do not violate non-signalling (that the reduced state of one system is invariant under operations on another) [4] . The standard version of box-world assumes there are only two binary outcome measurements under considerations. We label these X and Z and the outcomes ±1 in analogy with quantum theory. A normalized state can then, as discussed below, be represented as s =[‹ X › ‹ Z ›] T and is any mixture of the four extremal states [±1 ±1] T . The most general single system box-worlds are m -in n -out box-worlds, which mean that one selects one measurement setting from m possible settings and obtain n -valued outcomes. In particular, the 3-in 2-out box-world is the most analogous to a qubit in quantum theory. Expectation value representation For binary measurements, we find that focusing on the expectation values of measurements makes the notation very simple, and easy to visualize, along the lines of the example for box-world presented in Results. In what follows, we define a representation of states in terms of expectation values and relate it to the more standard representation in terms of probabilities, including showing that the transformations are matrices also in the new representation. Consider the case of states described in terms of two fiducial measurements with binary outcomes (recall that measurements are fiducial if their statistics are sufficient to determine the state). Such outcomes need not be normalized, but we require the sum of probabilities of both measurements to be equal. Consider the ‘probability’ representation of a state [4] : The following is the alternative (normalization-including) ‘expectation value representation’: where if the state is normalized n =1, and if it is subnormalized n <1. (For a subnormalized state we still use the notation ‹ g ›:= p ( g =+1)− p ( g =−1), implying the range − n ≤‹ g ›≤ n .) If a transformation T acts as a matrix on the state–vector in the probability representation, as it should if it respects mixtures, is it also a matrix in the expectation value picture? Suppose for the sake of argument that (i) there exists a fixed matrix M such that ν = M s for all states, (ii) the effective inverse matrix M −1 also exists satisfying M −1 M s = s ∀ s . Then we can write where ν ′ is the expectation representation state after the transformation. Thus, we see that if the two assumptions above hold then the state transformations by a matrix also in the expectation value picture. Moreover, these two assumptions do hold here, with (for example): The above argument naturally generalizes to more measurements. Note also that we could have used a different label for the positions in the probability picture (that is, not ±1) and then mapped that into the expectation value picture using the same matrix as above. In this sense, our argument does not depend on how we have labelled the two positions. Minimal representation of states Choosing a good representation of the states and transformations significantly aids the proof, and we shall therefore allow ourselves to introduce a third representation, intermediate between the expectation value and probability representations described above. We take a state in the probability representation and re-express it in the following way: where in the case of Z the different numbers are arbitrary labels for the different branches. For example, in the case of two branches and two fiducial measurements (labelling up=0 and low=1), the state would be expressed as Any state where all measurements have the same degree of normalization can be expressed in this representation, and one sees that there exists a matrix that maps states from the probability representation to this new one, as well as another matrix for the other direction. Thus, by the arguments made earlier, matrices representing transformations in the probability picture are also matrices in this new picture. For our purposes, the advantage of this new picture over the probability picture is that all parameters are independent, and the advantage over the expectation picture is that it is easier to express measurements with more than two outcomes. Proof of main theorem We restate our main claim for reference: Theorem: If the state space is a fully restricted conditional on the position measurement, then any non-classical transformation can always be localized to a strict subset of branches without violating branch locality. If the state space is instead fully independent of the position measurement then no non-classical transformations (of form T≠) can be localized to any strict subset of branches without violating branch locality. Proof : Recall that non-classical transformations are defined as phase transforms associated with the position measurement, that is, ’s such that where e z is an effect associated with an outcome of the position measurement, and η is a valid state [14] . Recall also the branch locality condition (Definition 1), that for a transformation , acting on a subset of branches , any state for which the inner product with the effect associated with the position being in , satisfies, , Let us consider first state spaces that are fully conditionally restricted with respect to the position measurement. In a fully conditionally restricted theory there is only one state corresponding to certain occupation of a given branch. Label the state corresponding to branch k certainly being occupied as , this is the unique state satisfying Any position phase transformation , moreover, preserves the position probability (equation 13). Thus, crucially, for all branches k and any phase transformation . This is precisely the branch locality condition for being localized to other branches than k , which means can be implemented on a strict subset of the branches without violating branch locality. This proves the first part of the main theorem. Now we consider state spaces that are fully independent of the position measurement. In this case, we will apply the branch locality condition of equation (14) where is any strict subset of branches, and show that this restricts the choice of phase transformation to . To prove this we will show that holds for sufficiently many linearly independent η such that they span the whole state space, implying . (Then a general vector ε can be written in terms of the linearly independent eigenvectors, such that every ε is left unchanged by : the very definition of an identity operation.) How many such eigenvectors are needed to span the full state space? We are considering many-branched interferometers, in which the position measurement Z can take two or more outcomes. We use the minimal representation of states defined in an earlier section in the Methods titled ‘Minimal representation of states’. Recall that each branch has at least one state where the Z statistics indicate that, if measured, the system will be found in that branch with certainty. There can also be additional X measurements, each with an arbitrary number (greater than one) of possible outcomes. In such cases, where the Z measurement has N possible outcomes the total number of degrees of freedom M from the other X measurements (each X i with m i different outcomes) is given by The total number of degrees of freedom in the state space (and hence the dimensions of the state vector in the minimal representation introduced above) is d = N + M . A transformation on the state can therefore be represented by a d × d matrix. We need d independent +1 eigenvectors η to prove that . We shall now identify these. Consider a transformation localized to a strict subset of branches, of size K where 1≤ K < N . If we pick some arbitrary η associated with one branch not in , because we will find a state that is subject to the branch locality restriction (equation 14). Because the state space is fully independent of the Z measurement, we can then freely alter each of the M degrees of freedom in X in turn (without altering the Z statistics), and thus can fully span all possibilities of X with an additional set of M linearly independent vectors. Each of these also satisfies the branch locality restriction, giving us M +1 independent vectors from one branch. Each of the remaining N − K −1 branches not in considered after this will then contribute one additional linearly independent state vector subject to branch locality. We thus find M + N − K independent state vectors associated with a +1 eigenvalue of . To identify the final K eigenvectors, we use the restrictions placed by requiring that preserves the position measurement statistics (equation 13). Let us pick K more states with arbitrary X statistics, each with support on a different branch in set , and labelled according to this choice of branch as η 1 to η K . These vectors are linearly independent of each other and the other M + N − K vectors we have found so far. Consider one of the vectors η i with support on branch . The most general form of the action of on this vector can be written as where are real numbers, and is a linear combination of the +1 eigenvectors without support in , which we found above. Let e b be the effect associated with measuring the position to be in branch , such that e b · η i =1 when b = i , and for all other branches where b ≠ i , e b · η i =0. As is a phase transformation, it must preserve for every branch b . By considering e i , we can thus conclude that , and similarly considering e j for all other branches in except i , we find that all other . We can thus re-express the action of as . Consider the repeated application of to the system. First note that , since is a linear combination of +1 eigenvectors of (the eigenvectors found from the branch locality condition). It then follows that after n applications of , . Valid transformations must take allowed states to allowed states, and so must be a valid state for all n (when is a valid state, applying must generate another valid state). This will only be the case for all n if (otherwise there will eventually be a measurement outcome with probability outside the allowed range of the theory). Thus for to be an allowed transformation, T η i = η i , such that η i is a +1 eigenvector of . An identical argument can be made for each of the K branches in , allowing us to find a set of K independent +1 eigenvectors from phase considerations. In total, we have found d = M + N linearly independent +1 eigenvectors of , showing that when considering the operations that are localized to some subset of branches in state spaces that are fully independent of the position measurement. This proves the second half of the theorem. Mutually unbiased measurements We can return to the definition of mutually unbiased measurements (Definition 5), and discuss it in more depth. We first consider what it means for one measurement to be unbiased with respect to another. Consider a measurement X with effects { x i } and measurement Y with effects { y i }. X is unbiased with respect to Y if for each permutation of the X outcome statistics, there will be a P x such that the total set of X outcomes, { x i · P x s } is equal to { x i · s }, and none of the Y outcomes are changed, such that y i · s = y i · P x y i for all y i , and further more P x s should be a valid state, and this should hold for all valid states s in the theory. Note that we do not require P x to be a physically allowed transformation—just an automorphism of the state space. The existence of some P x is required for the measurement to be part of a mutually unbiased set according to this definition. Furthermore, we note that the statistics associated with other measurements than Y do not have to be preserved. We then say a set of measurements is mutually unbiased if each measurement in the set is unbiased with respect to every other measurement in that set. By this definition, a set-up that can be entirely expressed by mutually unbiased measurements is symmetric under the relabelling of any of its measurement outcomes. We remark that this condition places a requirement on the state space as a whole rather than on individual states within it. A square gbit (with binary measurements X and Z ) could satisfy the above, but still admit ‘corner’ states such as (+1, +1) where both measurements are simultaneously known. This is because (+1, −1) and (−1, +1) are also allowed states, and so this more general definition still classifies X and Z as mutually unbiased. In contrast, X and Z in a ‘parallelogram’ bit (such that when Z =+1 the range X =[0, 1] is allowed, and when Z =−1 the range X =[−1, 0] is allowed; with all other allowed states chosen to form a convex set), would not be described as mutually unbiased, as it is not always permissible to exchange the outcomes of just the Z statistics. A further example is the following: consider a theory with three binary ±1 measurements, X , Y and Z where the outcomes of Y and Z are always the same. Writing a general state in the (normalized) expectation value picture as ( x , y , z ), if for every state, there is another valid state of the form ( x , − y , ?) and (− x , y , ? ), then X and Y form a mutually unbiased set. In the former case, ? becomes − z , and so the ‘permutation’ on Y has also affected the Z measurement, but this is allowed by the definition, as Z is not claimed to be within the set of mutually unbiased measurements. This set of unbiased measurements cannot be expanded to also include Z , as in general the state ( x , − y , z ) will not be valid, due to the restriction y = z . A set of mutually unbiased measurements that are fully conditionally restricted obey the quantum-like uncertainty relation. Consider a set of mutually unbiased measurements { X 1 , … X N } that are fully conditionally restricted. For such a set, when one measurement ( X i ) has an outcome that occurs with certainty, there will only be one allowed set of statistics for the rest of the measurements. From our definition of mutually unbiased measurements, one can always find a valid state associated with the statistics formed by any permutation of the outcomes of any of the mutually unbiased { X j } j ≠ i measurements. However, as there is only one valid set of statistics with the particular X i outcome, the statistics of every other X i measurement must be unchanged under any permutation. This is only true when all the outcome probabilities for a particular measurement have the same value, corresponding to the uniformly random distribution. Thus, a mutually unbiased set of measurements that are fully conditionally restricted will obey a quantum-like uncertainty principle. We now show how our definition reduces to the usual quantum definition of mutually unbiased bases in the quantum case: that for two measurements on a d -dimensional Hilbert space, X and Y , associated with d eigenstates {| x i ›} and {| y i ›}, respectively, X and Y are mutually unbiased if |‹ x i | y j ›| 2 =1/ d for all i and j . Consider projective measurements X and Y with d independent outcomes. It is possible to assume in quantum theory (for example, following a measurement) that we are in an eigenstate with respect to one of these measurements, and therefore states of the form ρ i =| x i ›‹ x i | are allowed. If we are in the eigenstate | x j › of X , the only allowed set of measurement statistics for Y is given by: Replacing | x j › with | x k ›, there will also be only one allowed set of Y statistics, given now by P ( Y = y i | X = x k )=|‹ y i | x k ›| 2 . By our definition, if X and Y are mutually unbiased measurements, the state in which we have permuted X without altering the Y statistics must be allowed. As there is only one set of Y statistics for the states | x j › and | x k ›, we therefore see that |‹ y i | x 1 ›| 2 =|‹ y i | x 2 ›| 2 = ⋯ =|‹ y i | x d ›| 2 for every i . Similar logic can be made for pure states of Y , such that |‹ x j | y 1 ›| 2 =|‹ x j | y 2 ›| 2 = ⋯ =|‹ x j | y d ›| 2 for each j . As |‹ x j | y i ›| 2 =|‹ y i | x j ›| 2 , this implies that this inner product squared is the same for every pair | x j ›, | y i ›. For a normalized Y measurement ∑ j |‹ x i | y j ›| 2 =1 for each pure state | x i ›, and we can replace the sum with any element in the sum repeated d times, such that d |‹ y i | x j ›| 2 =1 for all, i , j . Hence for all i and j , recovering the quantum definition for projective measurements X and Y to be mutually unbiased. How to cite this article: Dahlsten, O. C. O. et al . The uncertainty principle enables non-classical dynamics in an interferometer. Nat. Commun. 5:4592 doi: 10.1038/ncomms5592 (2014).